Genetic integration of local dispersal and exploratory behaviour in a wild bird Dispersal is a major determinant of the ecological and evolutionary dynamics of natural populations. Individuals differ greatly in the likelihood and distance of dispersal, but it is generally unclear to what extent intrinsic, possibly genetic, differences contribute. Here we present the first explicit empirical evidence for genetic coupling of local dispersal and exploratory behaviour, a key ‘animal personality’ trait. Using relatedness data from a multi-generation pedigree of free-living great tits ( Parus major ), we find quantitative genetic variation for both the distance of local dispersal within our study area and the rate at which individuals explore a novel environment. Moreover, we find a strongly positive genetic correlation between local dispersal distance and exploration rate, despite a weak and non-significant phenotypic correlation. These findings demonstrate a potentially important behavioural mechanism underlying heritable differences in local dispersal and highlight the potential for concerted evolution of dispersal and animal personality in response to selection. Dispersal—the movement of individuals from their place of birth to the place of breeding—is a key determinant of the ecological and evolutionary dynamics of natural populations [1] , [2] . In wild populations, individuals differ greatly in the likelihood and distance of dispersal [1] , [3] . Part of this variation can be explained by conditional dispersal behaviour in response to environmental cues such as rearing conditions, habitat quality and local population density [1] , [2] , [3] , [4] . However, it is generally less clear to what extent intrinsic, possibly genetic, differences among individuals also contribute [4] . In a world that is variable in both space and time, dispersal can increase the fitness of individuals, because it allows them to settle in new and potentially better breeding areas with, for example, fewer competitors, or higher-quality habitat or mating partners [1] , [2] . However, dispersing individuals may also face fitness costs, for example, because of increased mortality due to predation or starvation, and uncertainty of successful settlement elsewhere [1] , [2] . Dispersing individuals may express integrated dispersal phenotypes with distinct physiological, morphological, behavioural and/or life-history traits [5] . These so-called ‘dispersal syndromes’ [4] reduce the costs of dispersal and improve the chances of successful settlement elsewhere [1] , [6] . Recent theory suggests that individual variation in dispersal and other life-history traits may also be functionally integrated with variation in animal personality [4] , [7] , [8] , [9] . The general occurrence of animal personality variation [10] , [11] , [12] —individual differences in suites of correlated behaviours, which are consistent across time and different contexts [11] , [12] ; also often referred to as variation in temperament [11] or behavioural syndromes [12] —challenges the common notion that behaviour is largely plastic, which would allow individuals to respond optimally in any given situation. This realization has recently led to intense investigations into the adaptive significance [7] , [9] , as well as the ecological and evolutionary consequences [13] , [14] , of observed between-individual variation in basal behavioural traits, such as exploration, boldness, sociability and aggression [10] . A number of these studies, in various vertebrate taxa (including fish, lizards, birds and mammals), have reported phenotypic correlations between these personality traits, in particular exploratory behaviour, and dispersal tendencies (reviewed in Clobert et al. [4] and Cote et al. [8] ). However, whether dispersal and personality traits are also genetically correlated, thereby being constrained in their independent evolution, remains largely untested [4] , [8] . We investigate the quantitative genetic basis of local dispersal and exploratory behaviour, and tested for their genetic coupling, using data from a long-term population study of free-living great tits breeding in nestboxes in a mosaic landscape in the ‘Boshoek’ area in northern Belgium. The great tit presents possibly the best-studied example of a free-living animal with consistent and correlated between-individual behavioural variation [8] , [11] , [12] , [15] . Evidence from at least four populations across Western Europe, including the population investigated here, shows that individuals differ consistently in the rate at which they explore novel environments, measured in a standard behavioural test [16] . Previous investigations have found that fast-exploring individuals are also bolder when approaching novel objects and more aggressive towards conspecifics, compared with slow explorers (reviewed in Groothuis and Carere [15] ). The variation in exploration rate has a heritable component [17] , [18] , and phenotypic correlations have been reported between exploration rate and dispersal [19] , [20] , as well as spatial behaviour during foraging [21] , [22] . Here we test whether dispersal and exploratory behaviours are also genetically integrated by estimating the genetic correlation [23] between the distance of local dispersal within our study area and exploration rate. We used the quantitative genetic ‘animal model’ approach for estimating the additive genetic variances and covariance for local dispersal and exploration. The animal model allows for the use of relatedness information from complex multigenerational pedigrees to estimate quantitative genetic parameters, while controlling for potentially confounding effects (for example, because of relatives sharing the same environment) through the inclusion of additional random and fixed variables [23] , [24] . Here, using relatedness data from a 12-generation pedigree of the Boshoek great tit population, we find quantitative genetic variation for both the distance of local dispersal and the rate at which individuals explore a novel environment. Moreover, we find a strongly positive genetic correlation between local dispersal distance and exploration rate, despite a weak and non-significant phenotypic correlation. By showing the genetic integration of animal personality and local dispersal, we demonstrate a potentially important behavioural mechanism underlying heritable differences in local dispersal. Our findings further indicate that dispersing individuals may form a genetically non-random subset of the population and highlight the potential for concerted evolution of dispersal and animal personality in response to selection. Overview of local dispersal and exploration data The Boshoek great tit population has been intensively studied since 1994. Breeding attempts in nestboxes in 14 study plots ( Fig. 1 ) are routinely monitored, and all breeding adults and their offspring were captured and individually ringed. Approximately half of the breeding population consists of local recruits [25] . These data enabled us to construct (for details see Methods) a 12-generation deep social pedigree spanning 19 cohorts (born from 1991 to 2009), with 2,404 parent–offspring links informative to our analyses (1,219 maternal and 1,185 paternal links) ( Fig. 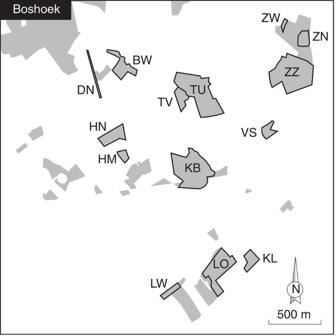Figure 1: Map of the Boshoek study area in Belgium. Woodlands are indicated in grey; the area between the woodlands mainly consists of agricultural land and some roads and scattered houses. The 14 study plots with nestboxes included in the analyses of local dispersal distance and exploration rate of great tits are indicated (for sample sizes per study plot seeSupplementary Table S1; figure made by Oscar Langevoord). 2 , Table 1 ). We estimated dispersal distances ( Fig. 3a ) within the study area for 1,230 individuals born from 1994 to 2009 as the shortest distance (in metres) from the location of birth to the location of first breeding, that is, ‘natal dispersal’ [1] , [19] (the maximum observed dispersal distance was 3,704 m; we could not measure larger dispersal distances of birds moving outside of the study area, hence we use the term ‘local dispersal’; for sample sizes per study plot see Supplementary Table S1 ). We measured the exploration rates ( Fig. 3b ) for 806 individuals captured in the field from 2005 to 2009 (individuals born from 2000 to 2009) following a standard test protocol [16] (for details see Methods; for sample sizes per study plot see Supplementary Table S1 ). Figure 1: Map of the Boshoek study area in Belgium. Woodlands are indicated in grey; the area between the woodlands mainly consists of agricultural land and some roads and scattered houses. The 14 study plots with nestboxes included in the analyses of local dispersal distance and exploration rate of great tits are indicated (for sample sizes per study plot see Supplementary Table S1 ; figure made by Oscar Langevoord). 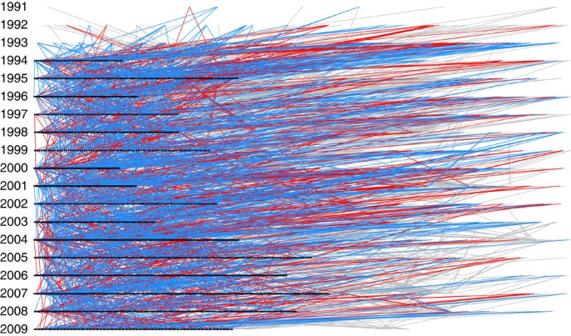Figure 2: Representation of the pedigree of the great tit population in Boshoek. Each line connects a parent with one of its offspring. Birth years of cohorts are indicated on the left. Parent–offspring links that are informative with regard to our quantitative genetic analyses of local dispersal and exploratory behaviour are indicated in colour (red and blue;N=2,404), and overlay the full population pedigree, which is indicated in grey. Red lines indicate maternal links (N=1,219); blue lines indicate paternal links (N=1,185). Black dots indicate individuals for which dispersal distance (N=1,230) and/or exploration rate (N=806) was measured (combined:N=1,818). The age of individuals born before 1994 was estimated based on plumage characteristics and previous ringing data in case of a small number of individuals. The pruned pedigree that is informative for our quantitative genetic analyses only includes individuals who have known phenotypes for dispersal distance and/or exploration rate and/or who are related to two or more phenotyped individuals. Full size image Figure 2: Representation of the pedigree of the great tit population in Boshoek. Each line connects a parent with one of its offspring. Birth years of cohorts are indicated on the left. Parent–offspring links that are informative with regard to our quantitative genetic analyses of local dispersal and exploratory behaviour are indicated in colour (red and blue; N =2,404), and overlay the full population pedigree, which is indicated in grey. Red lines indicate maternal links ( N =1,219); blue lines indicate paternal links ( N =1,185). Black dots indicate individuals for which dispersal distance ( N =1,230) and/or exploration rate ( N =806) was measured (combined: N =1,818). The age of individuals born before 1994 was estimated based on plumage characteristics and previous ringing data in case of a small number of individuals. The pruned pedigree that is informative for our quantitative genetic analyses only includes individuals who have known phenotypes for dispersal distance and/or exploration rate and/or who are related to two or more phenotyped individuals. Full size image Table 1 Statistics for the pruned pedigree of the Boshoek great tit population. 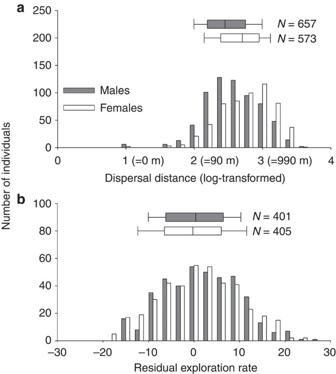Figure 3: Local dispersal and exploratory behaviour of great tits. Frequency distributions and box plots of the phenotypic data used in the animal model analyses: (a) local dispersal distance (totalN=1,230) and (b) exploration rate (totalN=806), for males and females separately. Dispersal distances (in metres) were10log(x+10) transformed; exploration rates are residuals from a linear regression on the date of the exploration test (from 1 July; see Methods). Boxes indicate the median, and 25th and 75th percentiles; whiskers indicate the 10th and 90th percentiles. Sample sizes are indicated in the graphs for males and females separately. Females dispersed significantly further than males (means±s.e.m. (in metres): males, 423±16; females, 631±22; F1,1228=70.17,P<0.001, analysis of variance (ANOVA), tested for10log(x+10) transformed data). The maximum observed distance was 3,704 m (=3.57 after log-transformation). There were no sex or age effects on exploration rates (allP>0.3, ANOVA). Full size table Figure 3: Local dispersal and exploratory behaviour of great tits. Frequency distributions and box plots of the phenotypic data used in the animal model analyses: ( a ) local dispersal distance (total N =1,230) and ( b ) exploration rate (total N =806), for males and females separately. Dispersal distances (in metres) were 10 log( x +10) transformed; exploration rates are residuals from a linear regression on the date of the exploration test (from 1 July; see Methods). Boxes indicate the median, and 25th and 75th percentiles; whiskers indicate the 10th and 90th percentiles. Sample sizes are indicated in the graphs for males and females separately. Females dispersed significantly further than males (means±s.e.m. (in metres): males, 423±16; females, 631±22; F 1,1228 =70.17, P <0.001, analysis of variance (ANOVA), tested for 10 log( x +10) transformed data). The maximum observed distance was 3,704 m (=3.57 after log-transformation). There were no sex or age effects on exploration rates (all P >0.3, ANOVA). Full size image Univariate animal models First, we fitted univariate animal models partitioning the phenotypic variance for local dispersal distance and exploration rate separately. These analyses demonstrated the presence of significant additive genetic variance for each trait, amounting to (narrow-sense [23] ) heritability estimates of h 2 =0.15±0.058 s.e. ( P =0.0036, log-likelihood-ratio test) and h 2 =0.30±0.11 s.e. ( P =0.0096, log-likelihood-ratio test) for local dispersal distance and exploration rate, respectively ( Fig. 4 ; Table 2a ). Natal brood identity also explained part of the variation in both local dispersal distance (6.7% of variance) and exploration rate (16.7% of variance), indicating an influence of parental and/or other common-environment effects at brood level (inclusion of a maternal or paternal effect instead of the natal brood effect resulted in similar results; Supplementary Tables S2 and S3 ). Birth plot and birth year effects explained only very small fractions of the variance in local dispersal distance and exploration rate (≤1.4% of variance; Table 2a ; Fig. 4 ). These results confirm previous reports of heritable variation for local dispersal distance [26] and exploration rate [17] , [18] estimated for other wild great tit populations. 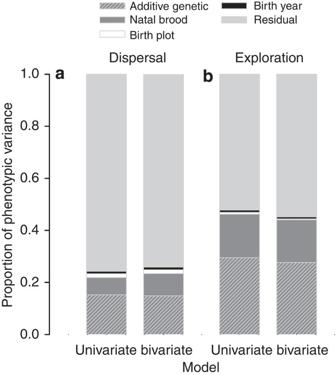Figure 4: Variance components for local dispersal distance and exploration rate of great tits. Relative contributions of variance components for (a) local dispersal distance and (b) exploration rate as derived from univariate animal models for each of the two traits separately, as well as from a single bivariate model. Additive genetic variances were significantly different from 0, indicating significant heritability for both traits (for details seeTable 2). Figure 4: Variance components for local dispersal distance and exploration rate of great tits. Relative contributions of variance components for ( a ) local dispersal distance and ( b ) exploration rate as derived from univariate animal models for each of the two traits separately, as well as from a single bivariate model. Additive genetic variances were significantly different from 0, indicating significant heritability for both traits (for details see Table 2 ). Full size image Table 2 Variance components for local dispersal distance and exploration rate in great tits. Full size table Bivariate animal model Next, we fitted a bivariate animal model that included both local dispersal distance and exploration rate as response variables to estimate the additive genetic covariance between the two traits. The bivariate model confirmed the estimates of variance components and heritabilities from the univariate models ( Fig. 4 ; Table 2b ). Moreover, the bivariate model demonstrated the presence of significant additive genetic covariance for local dispersal distance and exploration rate, resulting in a strongly positive genetic correlation of r G =0.99±0.40 s.e. ( P =0.0062, log-likelihood-ratio test; Table 2b ). Notably, the strong genetic correlation between local dispersal distance and exploration rate translated into a much weaker and non-significant phenotypic correlation between the two traits ( r P =0.074±0.064 s.e. ; P =0.39, log-likelihood-ratio test; estimated from residual variances and covariance when all other random terms were removed from the model). Spatial effects on local dispersal distance It is known that the measurement of local dispersal distances within a confined study area can potentially lead to a non-genetic resemblance in dispersal distance between parents and their offspring, as well as among siblings from the same brood, driven by the spatial configuration of the study area per se [27] . However, it is unlikely that such an effect generated spurious additive genetic variance for our dispersal data for the following reasons. First, the variance in local dispersal distance explained by birth plot was very small (1.4%, Fig. 4 , Table 2 ), indicating the large-scale spatial configuration of our study area to be unimportant in determining dispersal distance. Second, nestbox of birth explained <0.7% of the variance in local dispersal distance when included in the model ( Supplementary Table S4 ), also refuting the potential influence of small-scale spatial effects. Third, for each nestbox, we calculated the median distance to all potential destinations, defined as the end points of all recorded dispersal events in our data set. This covariate did not explain significant variation in local dispersal distance when included in our models ( P =0.47; F -test), and the estimates of quantitative genetic parameters remained qualitatively unchanged ( Supplementary Table S5 ). Finally, we used a simulation-based approach to assess the potential influence of the spatial configuration of the study area on the estimates of the heritability of local dispersal distance. We generated new dispersal data sets and associated pedigrees by randomly permuting nestboxes of origin (=birth) among the recruiting individuals within each cohort (for details see Methods). Although we found substantial variance due to plot effects in the analysis of the simulated data sets, the heritability estimates were very low (median=0.0095, upper 95% confidence limit=0.094) in comparison with the value of h 2 =0.15 for the real data estimated in the univariate model ( Table 2a ; Fig. 5 ). 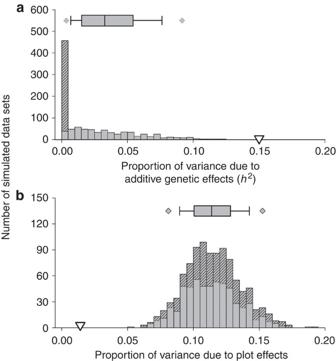Figure 5: Frequency distributions of variance components estimated for simulated dispersal data sets. The top panel (a) shows the distribution of heritability estimates (h2) for the simulated dispersal data sets (N=1,000); the lower panel (b) shows the distribution of estimates of the proportion of variance due to plot effects for these same data sets. Hatched bars indicate simulations for which the estimates of the additive genetic variance were bound to 0 (N=419). Boxes indicate the median, and 25th and 75th percentiles; whiskers indicate the 10th and 90th percentiles; and diamonds indicate the 5th and 95th percentiles. The triangles indicate the proportion of variance due to additive genetic (a) and plot effects (b) estimated from the observed dispersal data using a univariate animal model as reported inTable 2a; these estimates for the observed dispersal data fall outside the distribution of estimates for the 1,000 simulated data sets. For details on the simulation and model fitting approaches see Methods. Figure 5: Frequency distributions of variance components estimated for simulated dispersal data sets. The top panel ( a ) shows the distribution of heritability estimates ( h 2 ) for the simulated dispersal data sets ( N =1,000); the lower panel ( b ) shows the distribution of estimates of the proportion of variance due to plot effects for these same data sets. Hatched bars indicate simulations for which the estimates of the additive genetic variance were bound to 0 ( N =419). Boxes indicate the median, and 25th and 75th percentiles; whiskers indicate the 10th and 90th percentiles; and diamonds indicate the 5th and 95th percentiles. The triangles indicate the proportion of variance due to additive genetic ( a ) and plot effects ( b ) estimated from the observed dispersal data using a univariate animal model as reported in Table 2a ; these estimates for the observed dispersal data fall outside the distribution of estimates for the 1,000 simulated data sets. For details on the simulation and model fitting approaches see Methods. Full size image This study provides explicit evidence for the genetic coupling of local dispersal, an ecologically highly relevant trait, and exploratory behaviour, a trait that is increasingly used in widely diverging taxa to characterize animal personality variation [8] , [11] , [12] . Our results suggest that heritable variation in personality causes innate variation in individual dispersal tendencies, which may have a strong influence on the ecological and evolutionary dynamics of natural populations [13] , [14] . The contrast between the strong genetic and the much weaker phenotypic correlation that we found is a consequence of the modest heritabilities of both local dispersal distance and exploration rate and the negative (albeit non-significant) environmental (natal brood and residual) covariances between the two traits ( Table 2b ). The finding that the phenotypic correlation is substantially weaker than the underlying genetic correlation is not uncommon for behavioural traits [28] and further cautions against the use of phenotypic correlations for drawing inferences on the underlying genetic architecture of behavioural syndromes. At this point, the precise mechanism by which heritable variation in exploratory behaviour translates into heritable differences in local dispersal is still uncertain, because exploratory behaviour has been shown to associate with other personality traits, including boldness, risk-taking and aggression [11] , [12] , [15] . However, behavioural studies in our population have shown that exploration rate also predicts spatial patterns of foraging behaviour in non-territorial situations [21] , [22] , strongly suggesting that the genetic coupling between personality and local dispersal is driven by variation in innate exploratory tendencies rather than aggressive behaviour. This contrasts with previous findings in western bluebirds ( Sialia mexicana ), in which male dispersal propensity in an expanding population was genetically correlated with aggression [6] , [29] . More generally, our findings corroborate recent studies showing heritable variation for dispersal in several wild vertebrates (reviewed by Doligez and Pärt [30] ) and emphasize that individuals with longer dispersal distances may form a genetically non-random subset of the population, which has important implications for the study of fitness consequences of variation in dispersal as well as personality. Finally, our results indicate the potential of dispersal to evolve in response to selection, possibly through combined selection on genetically integrated behavioural and dispersal syndromes. General fieldwork The study was carried out using data from a wild population of great tits ( Parus major ) breeding in nestboxes in 14 study plots in the Boshoek area in Belgium (51°08′N, 4°32′E; Fig. 1 ). Since 1994, breeding attempts in nestboxes in the study area have been monitored through regular nestbox visits from April to June. Breeding adults and their nestlings are routinely captured inside their nestboxes and individually ringed. Standard biometry measures are taken, and body feathers are collected for DNA extraction. Individuals are sexed based on the presence (=female) or absence (=male) of an incubation patch or using molecular genetic markers [31] . Approximately half of the breeding birds are local recruits [25] , implying that if immigration and emigration are in equilibrium, approximately half of the surviving offspring emigrate out of the study area. Birds not ringed as nestlings in the study area are considered immigrants and are aged as either first-year or older birds based on plumage characteristics. For further details on the study site and general procedures during the fieldwork, see Nour et al. [32] and Matthysen [33] . Our study complies with legal requirements for research in Belgium. Permission for capture, transport and short-term housing of great tits was granted by the Belgian Ringing Scheme and the Flemish administration (‘Agentschap voor Natuur en Bos’). Pedigree We constructed a population pedigree by assigning the offspring of each brood to the male and female parent feeding it. Great tits normally breed in male–female pairs, with typically <10% of the offspring sired by extra-pair males [34] . A simulation study has previously shown that this level of extra-pair paternity causes only a minor bias in pedigree-based estimates of the additive genetic variance as derived from animal model methodology [35] . For a visual representation of the population pedigree see Fig. 2 ; for an overview of relevant pedigree statistics see Table 1 . The pedigree image and statistics were generated using the R [36] package PEDANTICS [37] . Local dispersal distance In our analyses of local dispersal distance, we only included individuals of known sex born in the study plots and years for which breeding attempts were monitored with equal intensity, and all breeding adults and their offspring were routinely captured and ringed (for sample sizes per study plot see Supplementary Table S1 ; see also Supplementary Fig. S1 ). We estimated local dispersal distances as the shortest distance (in metres) from the location of birth to the location of first breeding (that is, natal dispersal [19] ). Local dispersal distances (in metres) were 10 log( x +10) transformed before statistical analysis to improve the distribution of the residuals (using untransformed data gave similar results; Supplementary Table S6 , also see Supplementary Fig. S2 ). Exploration rate Free-living great tits were captured with mistnets around baited feeding tables or while sleeping in nestboxes. Captured individuals were transported to the laboratory where they were kept overnight and tested for exploration rate the following morning. Individual exploration rates were measured using a well-established protocol for testing exploratory behaviour in great tits [16] , [17] , [18] , [19] , [20] , [21] , [22] , which is an adapted version of the classical open-field test used for testing exploratory behaviour in rodents [38] . In brief, each bird was released in a test room with standard dimensions (4.0 × 2.4 × 2.3 m) containing five perches, after which the number of movements (hops and flights) was recorded during 2 min. The total number of movements during the 2-min period was taken as a measure of individual exploration rate. Individual exploration rates measured following such a protocol have previously been shown to be both repeatable and heritable [16] , [17] , [18] . Great tit exploration rates depend on the time of year [16] , [17] , and to control for this seasonal variation, we used residual exploration rates of the regression on test date (from 1 July; r =0.37, N =806, F 1,804 =130.47, P <0.001, F -test) in our analyses. Using raw exploration rates instead of residuals, while including exploration test date (from 1 July) as a covariate (fixed effect), in the models gave the same results ( Supplementary Table S7 ). We only included the first exploration test of individuals with known sex that were either born in one of the 14 study plots or immigrants into the study area ( N =806; Supplementary Table S1 , also see Supplementary Fig. S3 ). Animal models for estimating quantitative genetic parameters Using the pedigree information and phenotypic data on local dispersal and exploratory behaviour, we implemented univariate and bivariate animal models in the ASReml [39] software (version 3.0) partitioning the phenotypic variances ( V P ) for dispersal distance and exploration rate into their additive genetic ( V A ), natal brood identity ( V Brood ), birth plot ( V Plot ), birth year ( V Year ) and residual ( V R ) components, from which we calculated narrow-sense heritability ( h 2 ) estimates (as V A / V P ). Natal brood identity was included as a random effect ( V Brood ) to account for common-environment effects because of the shared early environment, including maternal and paternal effects, on the level of individual broods. Replacing the natal brood effect by either a maternal, paternal or nestbox effect gave similar results ( Supplementary Tables S2–S4 ). We used bivariate animal models to estimate the covariances for the additive genetic (COV A ), natal brood identity (COV Brood ) and residual (COV R ) terms, from which we calculated the additive genetic correlation ( r G ) between local dispersal and exploration (as COV A /√( V A, dispersal distance × V A, exploration rate ). In these bivariate models, the covariances for the birth plot and birth year terms were fixed at 0, because the very small fractions of variance explained by birth plot and year precluded a meaningful estimation of the covariances for these terms (although models actually estimating these covariances gave very similar quantitative genetic estimates; Supplementary Table S8 ). In all models, we included a fixed effect of sex on dispersal distance, to take into account sex differences in the distance of local dispersal (mean distance±s.e.m., in metres: males, 423±16; females, 631±22; F 1,1228 =70.17, P <0.001, analysis of variance, tested for 10 log( x +10) transformed data), which are general phenomena in birds [40] . There were no sex or age effects on exploration rates (all P >0.3, analysis of variance). Reported s.e. are as estimated by ASReml and should only be taken as indicative of statistical significance. We used log-likelihood-ratio tests to formally test for statistical significance of the random model terms (variances and covariances). Alpha was 0.05 for all analyses. Analyses of simulated dispersal data We used a simulation-based approach to investigate whether the spatial configuration of the study area could potentially generate additive genetic variance for dispersal distance by using the following procedure: first, we randomly permuted the nestboxes of origin (=birth) for all locally recruiting breeders ( N =1,230) on a per cohort basis. Based on the location of the randomly allocated ‘new’ birth nestboxes and the identity of their associated parent pairs, we then calculated new dispersal distances for all the recruits and constructed a new pedigree for each simulated dispersal data set. We chose to use this permutation method, because it is relatively straightforward to implement (for example, it does not require assumptions on the underlying distribution of dispersal distances and directions) while maintaining a data and pedigree structure similar to the original. We created a 1,000 simulated dispersal data sets and associated pedigrees. For each of these, we fitted an animal model including both an additive genetic ( V A ) and a birth plot ( V Plot ) effect to take into account the spatial configuration of the study area. Given that the simulations’ randomization procedure removes all structure from the data, except for the potential effects due to the spatial configuration of the area, it was not possible to fit more complicated models with additional effects, such as year effects, as the variances of these were bound to 0. These animal model analyses were run on the untransformed simulated dispersal distance data, because the simulated distance distributions were less skewed with average longer distances (average of the means: 1,150 m, for N =1,000 simulated data sets) than for the observed dispersal data (mean dispersal distance: 520 m, N =1,230 individuals). We do not consider this a problem for the analysis because a tendency for longer dispersal movements in the simulated data should actually increase the probability of finding spuriously high heritability estimates due to the spatial configuration of the study area. How to cite this article: Korsten, P. et al. Genetic integration of local dispersal and exploratory behaviour in a wild bird. Nat. Commun. 4:2362 doi: 10.1038/ncomms3362 (2013).